IL-37 protects against obesity-induced inflammation and insulin resistance Cytokines of the IL-1 family are important modulators of obesity-induced inflammation and the development of systemic insulin resistance. Here we show that IL-1 family member IL-37, recently characterized as an anti-inflammatory cytokine, ameliorates obesity-induced inflammation and insulin resistance. Mice transgenic for human IL-37 (IL-37tg) exhibit reduced numbers of adipose tissue macrophages, increased circulating levels of adiponectin and preserved glucose tolerance and insulin sensitivity after 16 weeks of HFD. In vitro treatment of adipocytes with recombinant IL-37 reduces adipogenesis and activates AMPK signalling. In humans, elevated steady-state IL-37 adipose tissue mRNA levels are positively correlated with insulin sensitivity and a lower inflammatory status of the adipose tissue. These findings reveal IL-37 as an important anti-inflammatory modulator during obesity-induced inflammation and insulin resistance in both mice and humans, and suggest that IL-37 is a potential target for the treatment of obesity-induced insulin resistance and type 2 diabetes. Obesity has reached epidemic proportions worldwide [1] and predisposes to the development of metabolic diseases, including type 2 diabetes and cardiovascular diseases. In obesity, adipocytes produce pro-inflammatory cytokines and chemokines [2] that can attract and activate macrophages [3] , [4] and other immune cells [5] , resulting in chronic low-grade inflammation [5] , [6] , [7] . The enhanced inflammatory status, illustrated by the production of pro-inflammatory cytokines, directly interferes with the insulin signalling pathway [8] , [9] , eventually leading to systemic insulin resistance and the subsequent development of type 2 diabetes [10] , [11] . Multiple pro-inflammatory cytokines have been identified that play a detrimental role in obesity-induced inflammation and insulin resistance, such as interleukin (IL)-1β and tumour necrosis factor-α (TNFα). However, cytokines that are able to restore the immunological misbalance in obesity have been less well studied. The IL-1 family consists of 11 members [12] , of which IL-1α, IL-1β, IL-1 receptor antagonist and IL-18 have been shown to play a pivotal role during obesity by modulating inflammatory responses [13] , [14] , [15] , [16] , [17] , [18] , [19] . Only recently has IL-1 family member IL-37, isolated in silico in the year 2000 (ref. 20 ), been identified for its anti-inflammatory actions by inhibiting innate responses [21] . During acute and chronic inflammation, IL-37 shifts the cytokine balance away from excessive inflammation [22] , thereby showing potency as a key factor to restore the inflammatory balance in obesity. The IL-37 gene has been mapped to chromosome 2 (ref. 23 ) and exists in five splice variants (IL-37a–e) [20] , [24] , [25] , [26] , [27] . IL-37b is the most complete variant containing five of the six exons and lacking a signal peptide. The IL-37 precursor contains a classic caspase-1 cleavage site, and caspase-1 processing appears to be required for nuclear translocation of IL-37 and its intracellular anti-inflammatory properties [28] , [29] . An instability element in exon 5 is known to control IL-37 messenger RNA expression. Subsequently, in the absence of inflammation, mRNA levels of IL-37 are rapidly degraded. In contrast, an inflammatory stimulus stabilizes IL-37 mRNA levels, thereby permitting its anti-inflammatory actions [30] . Previous studies have shown that IL-37 transgenic mice are protected from colitis [31] and lipopolysaccharide (LPS)-induced shock [21] . In the present study, we investigated whether IL-37 can counteract obesity-induced adipose tissue inflammation and protect against the development of insulin resistance. This was tested by examining adipose tissue samples from 80 humans for the expression of IL-37 and its relationship to inflammatory and metabolic markers. We also studied the effects of high-fat diet (HFD) in a unique human IL-37 transgenic mouse model and the in vitro properties of IL-37 on adipocyte function, insulin and AMPK signalling. We provide evidence for a role of IL-37 in ameliorating inflammation and insulin sensitivity in obesity. IL-37 is expressed in human adipose tissue First we evaluated the gene expression of IL-1 family members, including IL-37, in human adipose tissue in mature adipocytes (MAs) and stromal vascular cells (SVF) isolated from seven subjects. Whereas IL-1β, IL-1Ra and IL-18 showed higher expression in SVF, IL-37 was the only cytokine with higher mRNA levels in MA compared with SVF ( Fig. 1a ). mRNA analysis of paired adipose tissue samples of individuals demonstrated clear expression of IL-37 in adipose tissue, which was similar in visceral adipose compared with subcutaneous adipose tissue ( Fig. 1b ). In addition, western blot analysis revealed the presence of IL-37 in human adipose tissue at ~37 kDa ( Fig. 1c ). However, in adipose tissue IL-37 migrates at ~37 kDA, likely to be due to homodimerization, which was also reported elsewhere [21] . Moreover, the presence of IL-37 in human adipose tissue was confirmed by measuring the protein by a specific enzyme-linked immunosorbent assay ( Supplementary Fig. 1 ). 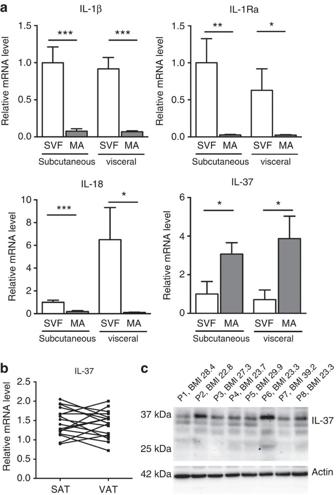Figure 1: IL-37 is expressed in human adipose tissue. Human adipose tissue was used to determine IL-37 expression. (a) mRNA levels of IL-1β, IL-1Ra, IL-18 and IL-37 in MA and SVF of subcutaneous and visceral adipose tissue,n=7. (b) mRNA levels of IL-37 in subcutaneous and visceral adipose tissue,n=17. (c) IL-37 was detected with western blotting analysis in human subcutaneous tissue,n=8. Error bars are shown as mean±s.e.m. *P<0.05, **P<0.01, ***P<0.001 (one-way analysis of variance). SVF, stromal vascular fraction; MA, mature adipocytes. Figure 1: IL-37 is expressed in human adipose tissue. Human adipose tissue was used to determine IL-37 expression. ( a ) mRNA levels of IL-1β, IL-1Ra, IL-18 and IL-37 in MA and SVF of subcutaneous and visceral adipose tissue, n =7. ( b ) mRNA levels of IL-37 in subcutaneous and visceral adipose tissue, n =17. ( c ) IL-37 was detected with western blotting analysis in human subcutaneous tissue, n =8. Error bars are shown as mean±s.e.m. * P <0.05, ** P <0.01, *** P <0.001 (one-way analysis of variance). SVF, stromal vascular fraction; MA, mature adipocytes. Full size image IL-37 reduces diet-induced obesity in mice To date, no complete mouse homologue for IL-37 has been found. Therefore, to examine the properties of IL-37 in a model of obesity in vivo , we employed a transgenic mouse strain expressing human IL-37 ( IL-37tg ) in all cells using a cytomegalovirus promoter [21] . The animals were fed High fat diet (HFD) (45% kcal derived from fat) or a control low-fat diet (LFD) (10% kcal derived from fat) for 16 weeks, and body weight gain and food intake were compared with wild-type (WT) animals ( Fig. 2a ). Starting body weight was similar between the WT and IL-37tg animals, yet body weight gain was significantly lower in HFD-fed IL-37tg mice compared with WT animals (−41% on HFD and −46% on LFD) ( Fig. 2b ), even though total caloric intake was similar in both genotypes ( Fig. 2c ). In line with lower body weight and epididymal white adipose tissue (WAT) mass ( Fig. 2d ), adipocyte size was smaller in the IL-37tg mice compared with WT animals ( Fig. 2e ), and paralleled by lower leptin ( Fig. 2f ) and strikingly higher plasma adiponectin levels ( Fig. 2g ). 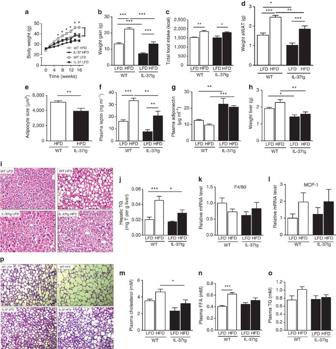Figure 2: IL-37 reduces diet-induced obesity in mice. IL-37tgand WT mice were fed an LFD or HFD for 16 weeks. (a) Body weight development and (b) body weight gain on LFD or HFD feeding. (c) Total caloric intake during 16 weeks of LFD or HFD. (d) Epididymal WAT (eWAT) weight after 16 weeks of LFD or HFD and (e) adipocyte size. Plasma concentrations of (f) leptin and (g) adiponectin after diet intervention. (h) Liver weights, (i) haematoxylin and eosin (H&E) staining of liver sections; magnification × 20 and (j) hepatic triglyceride (TG) content. qPCR analysis of macrophage infiltration markersF4/80(k) andMCP-1(i) in liver. (m) Plasma cholesterol, (n) free FAs and (o) triglycerides after 16 weeks of LFD or HFD. (p) H&E staining of brown adipose tissue; magnification × 20.n=10 mice per group. Error bars are shown as mean±s.e.m. *P<0.05, **P<0.01, ***P<0.001 (t-test or one-way analysis of variance). TG, triglycerides; FFA, free fatty acids. Figure 2: IL-37 reduces diet-induced obesity in mice. IL-37tg and WT mice were fed an LFD or HFD for 16 weeks. ( a ) Body weight development and ( b ) body weight gain on LFD or HFD feeding. ( c ) Total caloric intake during 16 weeks of LFD or HFD. ( d ) Epididymal WAT (eWAT) weight after 16 weeks of LFD or HFD and ( e ) adipocyte size. Plasma concentrations of ( f ) leptin and ( g ) adiponectin after diet intervention. ( h ) Liver weights, ( i ) haematoxylin and eosin (H&E) staining of liver sections; magnification × 20 and ( j ) hepatic triglyceride (TG) content. qPCR analysis of macrophage infiltration markers F4/80 ( k ) and MCP-1 ( i ) in liver. ( m ) Plasma cholesterol, ( n ) free FAs and ( o ) triglycerides after 16 weeks of LFD or HFD. ( p ) H&E staining of brown adipose tissue; magnification × 20. n =10 mice per group. Error bars are shown as mean±s.e.m. * P <0.05, ** P <0.01, *** P <0.001 ( t -test or one-way analysis of variance). TG, triglycerides; FFA, free fatty acids. Full size image IL-37 lowers liver and plasma lipids After HFD feeding, liver weight was lower in the presence of human IL-37 ( Fig. 2h ), which was paralleled by lower liver hepatic triglyceride content in HFD-fed IL-37tg mice as compared with WT animals ( Fig. 2j ) and by reduced levels of hepatic steatosis on HFD feeding, as visualized by haematoxylin and eosin staining ( Fig. 2i ). However, no significant differences were found in MCP-1 and F4/80 gene expression levels in the liver ( Fig. 2k,l ). Plasma cholesterol was significantly lower after HFD feeding in IL-37 animals compared with HFD-fed WT ( Fig. 2m ). Free fatty acid (FA) and triglyceride plasma levels in the animals showed similar tendencies towards lower values in IL-37tg animals compared with WT mice after the HFD intervention ( Fig. 2n,o ). To learn more about potential mechanisms that may explain lower body weight and amelioration in plasma lipid profile, we examined the brown adipose tissue, known to oxidize FAs for heat production. Owing to the large energy consumption, brown adipose tissue (BAT) highly contributes to plasma triglyceride clearance [32] . Although UCP-1 and PGC-1α levels were not altered in the IL-37tg mice compared with WT ( Supplementary Fig. 2a,b ), we observed a marked reduction in BAT lipid accumulation, in IL-37tg mice fed HFD compared with WT animals ( Fig. 2p ). IL-37 ameliorates diet-induced insulin resistance After HFD feeding, lower plasma insulin levels were observed in IL-37tg mice compared with WT mice, suggestive of preserved insulin sensitivity ( Fig. 3a ). Therefore, we performed an insulin tolerance test (ITT) and oral glucose tolerance test (oGTT). The ITT revealed that IL-37tg animals were partially protected against obesity-induced insulin resistance ( Fig. 3b ). In addition, the oGTT test demonstrated that IL-37tg animals had improved glucose tolerance on HFD feeding as compared with WT mice ( Fig. 3c ). 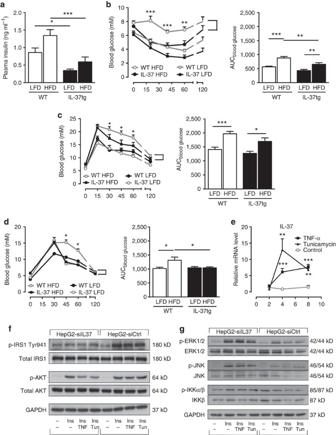Figure 3: IL-37 protects against obesity-induced insulin resistance. (a) Plasma insulin levels of mice after HFD.n=10 mice per group. (b) ITT test after 16 weeks of HFD (n=10 mice per group). (c) oGTT test after 16 weeks of HFD (n=10 mice per group). (d) oGTT test after 4 days of HFD (N=5 mice per group). (e) Time course in IL-37 mRNA levels in HepG2 cells exposed to TNF-α or tunicamycin (n=4). (f) Endogenous IL-37 was silenced using a siRNAs approach. Insulin receptor signalling was quantified by tyrosine (Tyr) 941 phosphorylation of the insulin receptor substrate 1 (IRS1) and phosphorylation of the downstream effector AKT. (g) Inflammatory kinases were blotted: ERK1/2, JNK and IKK α/β. Total amount of target protein and glyceraldehydes 3-phosphate (GAPDH) served as internal loading controls (n=4). Error bars are shown as mean±s.e.m. *P<0.05, **P<0.01, ***P<0.001 (one-way analysis of variance). AUC, area under the curve; Ins, insulin: 10 nM; TNF, tumour necrosis factor-α: 25 ng ml−1; Tun, tunicamycin 5 μg ml−1. Figure 3: IL-37 protects against obesity-induced insulin resistance. ( a ) Plasma insulin levels of mice after HFD. n =10 mice per group. ( b ) ITT test after 16 weeks of HFD ( n =10 mice per group). ( c ) oGTT test after 16 weeks of HFD ( n =10 mice per group). ( d ) oGTT test after 4 days of HFD ( N =5 mice per group). ( e ) Time course in IL-37 mRNA levels in HepG2 cells exposed to TNF-α or tunicamycin ( n =4). ( f ) Endogenous IL-37 was silenced using a siRNAs approach. Insulin receptor signalling was quantified by tyrosine (Tyr) 941 phosphorylation of the insulin receptor substrate 1 (IRS1) and phosphorylation of the downstream effector AKT. ( g ) Inflammatory kinases were blotted: ERK1/2, JNK and IKK α/β. Total amount of target protein and glyceraldehydes 3-phosphate (GAPDH) served as internal loading controls ( n =4). Error bars are shown as mean±s.e.m. * P <0.05, ** P <0.01, *** P <0.001 (one-way analysis of variance). AUC, area under the curve; Ins, insulin: 10 nM; TNF, tumour necrosis factor-α: 25 ng ml −1 ; Tun, tunicamycin 5 μg ml −1 . Full size image Acute effects of IL-37 on glucose tolerance To determine whether the beneficial effects of IL-37 on insulin sensitivity were independent of differences in body weight, we fed WT and IL-37tg animals a short-term HFD containing 60% kcal derived from fat for 4 days. The 4-day diet intervention did not affect body weight ( Supplementary Fig. S3 ). An oral GTT test revealed that the HFD-fed WT animals developed glucose intolerance as compared with the LFD-fed mice. In contrast, in the HFD-fed IL-37tg animals, glucose tolerance was preserved as compared with the mice receiving the LFD ( Fig. 3d ), suggesting that IL-37 directly ameliorates the adverse effects on glucose tolerance induced by chronic HFD feeding, and that this effect is independent of changes in body weight. We further assessed whether the improved glucose tolerance in the IL-37tg mice was due to differences in the insulin-producing β-cells. Islets were therefore stained for insulin and then mean staining intensity was measured as marker for insulin content. In IL-37tg mice, mean insulin staining intensity was lower compared with WT mice in both LFD- and HFD-fed mice ( Supplementary Fig. 4a ). In addition, islet hypertrophy was also observed in WT mice ( P =0.06 (one-way analysis of variance)). However, in IL-37tg mice, islet hypertrophy was not present ( Supplementary Fig. 4b,c ). Moreover, no differences were seen in the number of macrophages in the islets ( Supplementary Fig. 4d ). Together, these observations suggest preserved β-cell function and thereby improved metabolic control in IL-37tg mice after HFD. IL-37 directly improves insulin sensitivity We subsequently investigated the effect of IL-37 on insulin sensitivity using an in vitro approach. We revealed that silencing IL-37 hampers insulin signalling in human HepG2 cells that were stimulated with TNF-α or tunicamycin as inducers of insulin resistance [8] , [33] . Stimulation of these cells with either TNF-α or tunicamycin resulted in a significant increase of steady-state levels of IL-37 mRNA after 4 and 8 h ( Fig. 3e ). As shown in Fig. 3f , small interference RNA (siRNA)-mediated targeting to silence endogenous IL-37 (see Supplementary Fig. S5 ) significantly reduced activation of insulin receptor substrate 1 (IRS-1) as measured by tyrosine (Tyr) 941 phosphorylation. As a consequence, phosphorylation of the downstream effector molecule AKT was also reduced as compared with scrambled siRNA-treated cells. As shown in Fig. 3g , these differences could be partly explained by the increased activation of the inflammatory kinases ERK1/2, JNK and IKK α/β in cells silenced for IL-37. These kinases are known to cause insulin resistance via inhibition of the insulin signalling pathway, for example, by inhibition of IRS-1 (ref. 34 ). IL-37 downregulates the phosphorylation of these kinases as reported before [21] . IL-37 ameliorates diet-induced adipose tissue inflammation Furthermore, we investigated whether the IL-37tg mice were protected against HFD-induced adipose tissue inflammation, which may explain the improvement in insulin sensitivity. Therefore, we first investigated the adipose tissue of IL-37tg and WT mice for the presence of different immune cells using fluorescence-activated cell sorting (FACS) analysis of the stromal vascular fraction after 16 weeks of HFD feeding. Macrophage numbers were lower in IL-37tg mice (F4/80+CD11b+, −20%, P <0.05 ( t -test); Fig. 4a ). Similar reductions of other pro-inflammatory cells were observed for NK cells (NK1.1+, −46%, P <0.05 ( t -test); Fig. 4b ) and cytotoxic T cells (CD3+CD8+, −32%, P <0.05 ( t -test); Fig. 4c ), whereas there was no change in the amount of regulatory T cells (CD3+CD4+, nonsignificant ( t -test); Fig. 4d ) in the IL-37tg animals compared with WT animals fed the HFD. The reduction in pro-inflammatory status of the adipose tissue in the presence of IL-37 was confirmed by quantitative PCR (qPCR) analysis for various macrophage markers. F4/80 , CD11c and MCP-1 gene expression levels were all substantially lower in HFD-fed IL-37tg mice when compared with WT mice ( Fig. 4e–g ). In line with these data, immunohistochemistry demonstrated a reduced number of F4/80+ cells in the adipose tissue of IL-37tg mice ( Fig. 4i ) and a reduced amount of crown-like structures as compared with WT mice fed the HFD ( Fig. 4h ). Next, we further explored whether recIL-37 limits adipose tissue inflammation in Ob/Ob mice, an established obese mouse model with enhanced adipose tissue inflammation. Therefore, Ob/Ob mice were treated intraperitoneally with recIL-37 for 2 weeks. IL-1β levels were robustly reduced (−93%, P <0.01 ( t -test)), as was the secretion of pro-inflammatory IL-6 and CXCL1 in WAT of animals treated with recIL-37, as compared with animals receiving vehicle only ( Fig. 4j–l ). Moreover, similar changes were seen in mRNA expression of these cytokines, although the treatment did not change the number of macrophages that were present in the adipose tissue ( Supplementary Fig. 7 ). 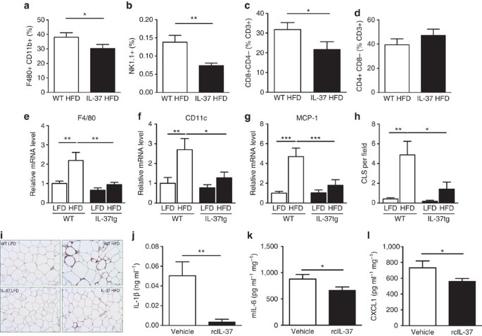Figure 4: IL-37 reduces infiltration of macrophages and lymphocytes into WAT. (a) Macrophages (F4/80+CD11b+), (b) NK cells (NK1.1+), (c) cytotoxic T cells (CD3+CD8+CD4−) and (d) regulatory T cells (CD3+CD4+CD8−), measured with flow cytometry. qPCR analysis of macrophage markers, (e)F4/80, (f)CD11c, (g)MCP-1in epididymal WAT (eWAT) of WT and IL-37tg mice following HFD for 16 weeks. (h) Macrophage influx into adipose tissue as determined by immunohistochemistry, F4/80 staining; × 20 magnification and (i) mean crown-like structures per image. Ob/ob mice were injected intraperitoneally with 1 μg per mouse per 2 days. Intracellular IL-1β (j) and excreted IL-6 (k) and CXCL1 (l) were significantly lower in recIL-37-treated mice.n=4 mice per group for microanalysis, for cytometryN=5, otherwisen=10 mice per group. Error bars are shown as mean±s.e.m. *P<0.05, **P<0.01, ***P<0.001 (t-test or one-way analysis of variance). CLS, crown-like structures. Figure 4: IL-37 reduces infiltration of macrophages and lymphocytes into WAT. ( a ) Macrophages (F4/80+CD11b+), ( b ) NK cells (NK1.1+), ( c ) cytotoxic T cells (CD3+CD8+CD4−) and ( d ) regulatory T cells (CD3+CD4+CD8−), measured with flow cytometry. qPCR analysis of macrophage markers, ( e ) F4/80 , ( f ) CD11c , ( g ) MCP-1 in epididymal WAT (eWAT) of WT and IL-37tg mice following HFD for 16 weeks. ( h ) Macrophage influx into adipose tissue as determined by immunohistochemistry, F4/80 staining; × 20 magnification and ( i ) mean crown-like structures per image. Ob/ob mice were injected intraperitoneally with 1 μg per mouse per 2 days. Intracellular IL-1β ( j ) and excreted IL-6 ( k ) and CXCL1 ( l ) were significantly lower in recIL-37-treated mice. n =4 mice per group for microanalysis, for cytometry N =5, otherwise n =10 mice per group. Error bars are shown as mean±s.e.m. * P <0.05, ** P <0.01, *** P <0.001 ( t -test or one-way analysis of variance). CLS, crown-like structures. Full size image To further understand the molecular pathways affected by IL-37 during development of obesity, a microarray analysis of the whole adipose tissue from HFD-fed WT and IL-37tg animals was performed. Hierarchical clustering of the microarray results led to a distinct separation of WT versus IL-37tg animals fed the HFD for 16 weeks ( Supplementary Fig. S8 ). Compared with the WT mice, 1,125 genes were significantly upregulated and 793 genes were downregulated in the adipose tissue of the IL-37tg animals ( P <0.01). 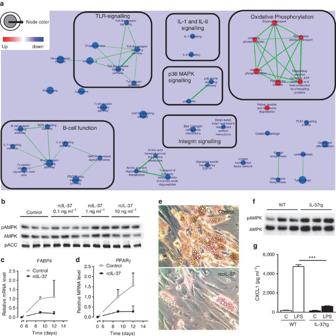Figure 5: IL-37 affects energy metabolism and AMPK activation. (a) Relevant and important differentially regulated pathways as identified by microarray analysis. (b) Murine 3t3 adipocytes were stimulated 1 h with recIL-37 and phospho-AMPK, AMPK and ACC levels were measured. Human SGBS cells were differentiated into adipocytes with or without recIL-37, and gene expression levels of (c)FABP4and (d)PPARγwere quantified. (e) Visualization of differentiated SGBS-cells with light microscopy (magnification × 20). (f) Bone marrow was differentiated into macrophages and levels of pAMPK and AMPK were determined. (g) Bone marrow-derived macrophages (BMDMs) were treated with LPS for 24 h and CXCL1 levels in medium were measured. Error bars are shown as mean±s.e.m. *P<0.05, **P<0.01, ***P<0.001 (one-way analysis of variance). Figure 5a shows the pathways that were regulated significantly different in the IL-37tg mice compared with WT mice, when analysed using Cytoscape. In the adipose tissue of the IL-37tg animals, several immune and inflammatory pathways including Toll-like receptor (TLR) signalling were downregulated compared with the WT mice. In line with downregulation of TLR signalling pathways, qPCR analysis of TLR-2 and TLR-4, known to mediate obesity-induced adipose tissue inflammation [35] , [36] , [37] , [38] , revealed reduced expression levels of both TLRs in adipose tissue of HFD-fed IL-37tg animals as compared with WT mice ( Supplementary Fig. S9b,c ). Noticeably, expression levels of TLR-1 increased similarly in both genotypes ( Supplementary Fig. S9a ). Figure 5: IL-37 affects energy metabolism and AMPK activation. ( a ) Relevant and important differentially regulated pathways as identified by microarray analysis. ( b ) Murine 3t3 adipocytes were stimulated 1 h with recIL-37 and phospho-AMPK, AMPK and ACC levels were measured. Human SGBS cells were differentiated into adipocytes with or without recIL-37, and gene expression levels of ( c ) FABP4 and ( d ) PPARγ were quantified. ( e ) Visualization of differentiated SGBS-cells with light microscopy (magnification × 20). ( f ) Bone marrow was differentiated into macrophages and levels of pAMPK and AMPK were determined. ( g ) Bone marrow-derived macrophages (BMDMs) were treated with LPS for 24 h and CXCL1 levels in medium were measured. Error bars are shown as mean±s.e.m. * P <0.05, ** P <0.01, *** P <0.001 (one-way analysis of variance). Full size image In addition, the microarray data revealed upregulation of a cluster of genes related to mitochondrial and oxidative phosphorylation in adipose tissue of HFD-fed IL-37tg animals as compared with WT mice, suggesting that IL-37 may directly influence specific metabolic pathways. IL-37 affects AMPK activation in macrophages and adipocytes Although AMPK is a central regulator of cellular metabolism [39] , its activation also results in several anti-inflammatory effects, for example, by reduced production of pro-inflammatory cytokines in response to LPS [40] . Activation of AMPK is known to have profound effects on adipose tissue, including anti-obesity effects [41] . In related studies, transfection of THP-1 cells with IL-37 resulted in >40% increase in phosphorylation of AMPK associated with a >60% reduction in mammalian target of rapamycin [21] . Therefore, we subsequently evaluated whether IL-37 affects AMPK signalling in adipocytes. Murine adipocytes were treated with recombinant IL-37 precursor IL-37 for 1 h and phosphorylation of AMPK was subsequently measured. Adipocytes that were stimulated with recIL-37 displayed increased phosphorylation of AMPK ( Fig. 5b ), revealing that IL-37 activates AMPK signalling. In addition, the activity of ACC, an important downstream target of AMPK, was also increased by recIL-37 treatment ( Fig. 5b ). Furthermore, Sestrin 2 , an important activator of AMPK, was increased in the presence of IL-37 in the HFD mice, suggesting a possible explanation by which AMPK activity was increased ( Supplementary Fig. 10 ). As activation of AMPK is known to potently inhibit adipocyte differentiation [42] , adipocytes from WT mice were subsequently differentiated in the presence of recIL-37, and mRNA levels of lipogenic genes PPAR γ and FAPB4 were measured. Indeed, recIL-37-treated cells displayed reduced adipocyte differentiation as indicated by reduced mRNA expression of FABP4 and PPARγ ( Fig. 5c,e ). In bone marrow-derived macrophages (BMDMs) from IL-37tg animals, pAMPK levels were elevated compared with WT mice ( Fig. 5f ) paralleled by reduced levels of CXCL1 secreted from these cells after LPS ( Fig. 5g ). These data show that AMPK is a key protein downstream of IL-37 signalling. IL-37 in human adipose tissue relates to insulin sensitivity Although IL-37 is present in adipose tissue [43] , its role in controlling inflammation in subjects with obesity and/or insulin resistance remains unknown. Therefore, we determined IL-37 levels in subcutaneous adipose tissue samples obtained from a cohort of 80 subjects with varying levels of body mass index (BMI), insulin sensitivity and degree of adipose tissue inflammation. We compared log-normalized levels of IL-37 gene expression values in human adipose tissue with adipose tissue leptin levels, the homeostatic model for insulin resistance (HOMA-IR) and markers of adipose tissue inflammation. IL-37 gene expression levels in adipose tissue were significantly higher in subjects with lower leptin protein levels ( Fig. 6a ). BMI was not associated with IL-37 mRNA levels in adipose tissue ( Fig. 6b ). We investigated whether the inflammatory status of the adipose tissue, as quantified by the level of macrophage infiltration, was associated with IL-37 expression. Indeed, the number of CD68-positive cells in adipose tissue was inversely associated with IL-37 mRNA expression levels ( Fig. 6c ). IL-37 expression was associated with improved insulin sensitivity, as determined by the HOMA-IR, such that individuals with a low HOMA-IR exhibited higher IL-37 mRNA levels in adipose tissue compared with persons with a higher HOMA-IR ( Fig. 6d ). Lastly, and in line with these findings, higher insulin levels were associated with lower IL-37 mRNA levels, whereas plasma glucose levels were not related to IL-37 adipose tissue expression levels ( Supplementary Fig. S11a,b ). 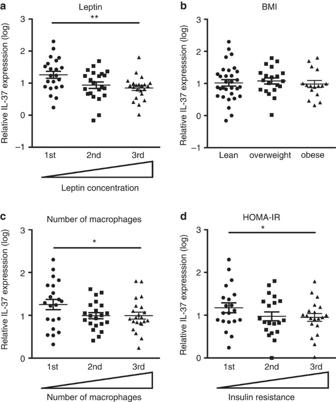Figure 6: IL-37 in humans. Steady-state IL-37 mRNA levels were determined in human subcutaneous adipose tissue of 80 subjects. (a) IL-37 mRNA expression in tertiles for adipose tissue leptin concentration and (b) in lean, overweight and obese subjects. (c) IL-37 mRNA expression in adipose tissue with tertiles for number of CD68+ cells and (d) IL-37 mRNA expression in persons with tertiles for HOMA-IR. Error bars are shown as mean±s.e.m. *P<0.05, **P<0.01, ***P<0.001 (one-way analysis of variance). BMI, body mass index; HOMA-IR, homeostatic model of insulin resistance. Figure 6: IL-37 in humans. Steady-state IL-37 mRNA levels were determined in human subcutaneous adipose tissue of 80 subjects. ( a ) IL-37 mRNA expression in tertiles for adipose tissue leptin concentration and ( b ) in lean, overweight and obese subjects. ( c ) IL-37 mRNA expression in adipose tissue with tertiles for number of CD68+ cells and ( d ) IL-37 mRNA expression in persons with tertiles for HOMA-IR. Error bars are shown as mean±s.e.m. * P <0.05, ** P <0.01, *** P <0.001 (one-way analysis of variance). BMI, body mass index; HOMA-IR, homeostatic model of insulin resistance. Full size image Adipose tissue inflammation is a key process in the development of obesity-induced insulin resistance. We demonstrate here that IL-1 family member IL-37 counteracts the detrimental effects of HFD feeding on weight, adipose tissue inflammation and systemic insulin resistance in IL-37tg mice. Moreover, treatment with recIL-37 in vivo and in vitro represses adipose tissue inflammation. We also report data suggestive of a similar function in human subjects. Together, these findings identify IL-37 as a potential new target to tackle obesity-induced insulin resistance and type 2 diabetes. First, these conclusions are based on the observations that transgenic mice expressing human IL-37 show a reduction in weight gain, lower adipocyte mass and size, less adipose tissue inflammation and less insulin resistance in response to HFD feeding in comparison with WT mice fed the same diet. Second, as IL-37tg mice show greater glucose tolerance after short-term feeding, the effect of IL-37 is weight-independent. Third, IL-37 preserves IRS-1 tyrosine (Tyr) 941 phosphorylation, thereby rescuing downstream insulin signalling. Fourth, IL-37 expression in human adipose tissue is inversely correlated with adipose tissue inflammation and the presence of insulin resistance. Thus, these data support a link between IL-37 biology, adipose tissue inflammation and insulin sensitivity. As food intake was similar between IL-37tg and control animals, other mechanisms probably underlie the decreased weight gain in IL-37tg animals during HFD-induced obesity. Interestingly, the microarray data revealed that oxidative phosphorylation and respiratory activity in WAT of the IL-37tg animals were increased compared with WT animals fed the HFD. Moreover, we show that IL-37 directly activates AMPK signalling and reduces adipocyte differentiation. This is in line with earlier described findings that overexpression of IL-37 in THP-1 cells increases AMPK and decreases mammalian target of rapamycin levels [21] . Moreover, other anti-inflammatory agents induce AMPK activation [44] . The increase of AMPK was accompanied by an increased ACC activity, providing evidence that IL-37 can activate metabolic pathways in adipocytes. It suggests the involvement of AMPK activation in the protecting effects of IL-37 against adipose tissue expansion on HFD feeding. Interestingly, recent data revealed that IL-18 signalling enhances FA oxidation via activation of AMPK signalling [45] . As both IL-37 and IL-18 bind to the same IL-18 receptor α chain (IL-18rα) [24] , our findings suggest that IL-37 can activate AMPK signalling via similar mechanisms, leading to increased FA oxidation and alleviation from development of obesity. Consistent with this observation, an enhanced activity of BAT may partly explain the protection against the development of obesity in IL-37tg animals. Importantly, IL-37 transgenic animals displayed markedly reduced adipose tissue inflammation, illustrated by reduced pro-inflammatory immune cell infiltration into the adipose tissue, as demonstrated by FACS analysis, qPCR and immunohistochemistry. Moreover, treatment of severely obese mice with recIL-37 reduced adipose tissue cytokine secretion, independent of body weight. In macrophages, the IL-37-dependent activation of AMPK may be aimed at counterbalancing pro-inflammatory actions. It has been previously shown that activation of AMPK in macrophages by 5-amino-1-β-D-ribofuranosyl-imidazole-4-carboxamide (AICAR), specifically inhibits pro-inflammatory cytokine production on LPS treatment [40] . Through its activation of AMPK, IL-37 may also directly inhibit inflammatory actions of immune cells. An alternative mechanism for the reduced obesity-induced inflammation is provided by our microarray analyses, showing downregulation of TLR signalling in IL-37tg mice after HFD. An inhibitory effect of IL-37 on TLR signalling in the IL-37tg mice would be consistent with a reduced ability to respond to FFA’s via triggering of TLR-2 or TLR-4 (refs 35 , 36 , 37 , 38 , 46 ) that can lead to macrophage activation [47] . Previous findings have shown that IL-37 is a fundamental inhibitor of the response to LPS [21] . Thus, during HFD-induced inflammatory cell infiltration into the adipose tissue, a comparable mechanism may be activated in the presence of IL-37. Through its anti-inflammatory properties, IL-37 not only reduces levels of pro-inflammatory cytokines but also prevents excessive immune cell activation in adipose tissue [21] . A probable molecular mechanism through which IL-37 exerts its anti-inflammatory effects is binding to the IL-18rα [24] , [48] . There are also data that demonstrate that exploitation of the properties of single immunoglobulin IL-1R-related protein and IL-18rα are both necessary for the protective effects of IL-37 (ref. 49 ). Single immunoglobulin IL-1R-related protein engagement is known to negatively regulate TLR and IL-1 signalling [50] , and may also explain IL-37 inflammation-dampening effects in adipose tissue. Indeed, the microarray data revealed that IL-37 acts as an inhibitor of TLR and IL-1-mediated pathways, which confirms earlier findings [21] . Besides extracellular binding, IL-37 has been shown to translocate to the nucleus where it may act as a transcriptional modulator [28] , as is the case with nuclear translocation of another member of the IL-1 family member IL-1α [51] , [52] . Altogether, these mechanisms probably account for the anti-inflammatory actions of IL-37 in the adipose tissue. The reduction of body weight and subsequent local inflammation may also account for the markedly enhanced adiponectin levels measured in the transgenic animals, as higher adiponectin levels are generally observed in lean individuals [53] . Conversely, more inflammation is associated with lower adiponectin levels [54] . In humans, we found that IL-37 expression in adipose tissue was inversely related to HOMA-IR. In the animal model, the presence of IL-37 protected against the detrimental effects on glucose tolerance and insulin sensitivity after HFD feeding. The effects of IL-37 appear independently of body weight changes, as IL-37tg animals were also protected against glucose intolerance on short-term HFD feeding that did not affect weight in either group. Moreover, we showed that IL-37 can preserve insulin sensitivity in vitro , by preserving phosphorylation of IRS-1 and downstream Akt for insulin signalling, via inhibition of inflammatory kinases JNK, ERK and IKKα/β that cause inhibitory serine phosphorylation of the insulin receptor substrate-1 (ref. 34 ). In addition, similar to IL-1 and IL-18 (refs 55 , 56 , 57 ), IL-37 affects the function of the insulin-producing β-cells. It is known that obesity can lead to islet hypertrophy and increased insulin secretion [58] , [59] , [60] . We showed that the presence of IL-37 spared pancreatic islets from hypertrophy and excessive insulin production, compared with WT mice. Overall, these findings reveal a role for IL-37 in determining insulin sensitivity. Inversely, reduced production of IL-37 may contribute to the onset of insulin resistance as absence of IL-37 may promote inflammation that directly interferes with insulin signalling routes. Currently, regulation of IL-37 expression or its mRNA stability in human adipose tissue is unknown. Interestingly, IL-37 mRNA expression is found in the adipocyte fractions of human adipose tissue, suggesting that adipocytes are sensitive for stimuli that induce IL-37 production. Repeated high levels of postprandial free FAs probably serve as triggers for IL-1 expression [61] and may also regulate IL-37 expression in adipose tissue. The co-expression of IL-37 next to IL-1 is therefore probably aimed at counterbalancing inflammation during obesity. As humans reveal an inverse correlation between inflammation in adipose tissue and expression of IL-37, it is likely to be that subjects who fail to express sufficient IL-37 locally will develop higher levels of inflammation. All in all, our findings show that IL-37 is important during the development of obesity by counteracting adipocyte differentiation, HFD-induced adipose tissue inflammation and insulin resistance. Moreover, increased IL-37 expression in human adipose tissue is associated with enhanced insulin sensitivity and a reduction in adipose tissue inflammation. IL-37 may therefore be a target to mitigate the detrimental effects of obesity, including type 2 diabetes mellitus. Human subjects Subcutaneous and visceral adipose tissues were obtained from healthy donors. Characteristics of donors are listed in Table 1 . For associations of IL-37 expression, subjects from the same CONTROL cohort were used. The total number of individuals in the control cohort was 80. Some measurements were not carried out in all subjects. Leptin was measured in n =66 subjects, BMI in n =47 subjects, CD68+ cells per 1,000 adipocytes in n =52 subjects and HOMA-IR in n =61 subjects. All subjects gave informed consent. The studies were approved by the ethical committee of the Radboud University Medical Centre, Nijmegen. Table 1 Subject characteristics of human adipose tissue biopsies (values are mean±s.d.). Full size table Mice IL-37tg mice on a C57Bl/6 background have been reported [21] . WT C57/Bl6 animals were purchased from Jackson Laboratories. All animal procedures were conducted under protocols approved by the animal experimentation committee of Radboud University Medical Centre, Nijmegen. Body weight of the animals was recorded weekly. Twenty male mice per genotype (10 weeks of age at the start of the dietary intervention) were used in the 16-week diet-intervention experiment. After a 2-week run-in period on LFD, mice were given LFD or HFD diet for 16 weeks, containing 10 or 45% kcal derived from fat, respectively (D12450B or 12451, Research Diets, Inc.). To investigate whether IL-37 had a body weight-independent effect, we performed a 1-week short-term high-fat study using a diet containing 60% kcal derived from fat (D12492, Research Diets). For this, ten male mice per genotype were used (12 weeks of age at the start of the intervention). Studies on glucose homeostasis At the end of diet-intervention study, oGTT and ITT tests were performed. Before the oGTT test, all 40 male animals were fasted overnight and 2 g kg −1 glucose ( D -glucose, Gibco, Invitrogen) was orally administered. Before the ITT test, mice were fasted 6 h and insulin (0.75 U kg −1 ) was injected intraperitoneally. Blood glucose levels were determined with an Accu-chek glucosemeter (Roche Diagnostics, Almere, The Netherlands) at stated time points. Cytokine measurements Plasma concentrations of insulin (Crystal Chem Inc., IL, USA), adiponectin, leptin (both R&D Systems, Minneapolis, MN, USA) were measured by ELISA. Leptin levels in human adipose tissue were measured with Milliplex (Millipore, Billerica, MA, USA). IL-37 protein levels were measured to determine levels in adipose tissue (R&D Systems). Histology/immunohistochemistry Morphometry of individual fat cells was assessed using digital image analysis. Microscopic images were digitized in 24-bit RGB (specimen level pixel size 1.28 × 1.28 μm 2 ). Recognition of fat cells was initially performed by applying a region-growing algorithm on manually indicated seed points, and minimum Feret diameter was calculated. For detection of macrophages/monocytes, an F4/80 antibody (Serotec, Puchheim, Germany) was used. Visualization of the complex was done using 3,3′-diaminobenzidine for 5 min. Negative controls were used by omitting the primary antibody. Haematoxylin and eosin staining of sections was done using standard protocols. Crown-like structures were counted with a microscope at a magnification of × 20, at least four images per sample. Human macrophages were visualized using CD68. The paraffin-embedded pancreas sections (5 μm) were deparaffinized/rehydrated in Clearene (Surgipath, IL, USA) followed by ethanol and PBS serial rehydration. Antigen retrieval was completed in citrate buffer, pH 6.0, for 15 min using a steamer, and sections were blocked with CAS-BLOCK solution (Invitrogen, NY, USA) for 1 h. Sections were then stained with guinea pig anti-insulin antibody (1:600, Dako Cytomation, Glostrup, Denmark) and incubated overnight at 4 °C. Cy3-conjugated donkey-anti-guinea pig IgG (1:200, Jackson Immunoresearch, West Grove, PA, USA) was used as a secondary antibody and incubated for 2 h at 25 °C. Counterstaining was performed with 5 μg ml −1 4',6-diamidino-2-phenylindole (Sigma, Rehovot, Israel). Next, slides were mounted with PermaFluor aqueous mounting medium (Thermo Scientific, MA, USA). Images were captured using an Olympus BX60 microscope. At least 30 islets were selected at random and analysed using the CellProfiler software, version 2.0. Mean fluorescent intensity was calculated by dividing the total staining intensity of each islet by its area. For quantification of the islet area, β-cells were visualized by an immunohistochemical approach using an antibody against insulin (sc9168, Santa Cruz Biotechnology, Heidelberg, Germany). Quantification was performed using ImageJ software (version V1.47t). A total of n =10 animals per group per genotype were analysed. Lipids Cholesterol, triglycerides and glucose (Liquicolor, Human GmbH, Wiesbaden, Germany) and free FAs (NEFA-C, WAKO Chemicals, GmbH, Neuss, Germany) were measured enzymatically following the manufacturers’ protocols. FACS analyses After washing with DMEM+0.1% BSA and FACS buffer (PBS+1% BSA), the stromal vascular fraction was extracted from the epididymal mouse WAT or human adipose tissue by digestion with 0.02% collagenase type 1 (Gibco, Invitrogen on HBSS containing 2% FA-free BSA) for 1 h. Cells were filtered with a 100-μM filter and centrifuged at 200 g for 10 min. Floating MAs were discarded and SVF was resuspended in erythrocyte lysis buffer (BD Pharmingen) for 10 min. Cells were washed twice with FACS buffer. Cells were divided into two equal parts and incubated with fluorescently labelled antibodies, including CD45-ECD (Coulter), CD3-APC (BD Pharmingen), CD4-FITC (BD Pharmingen), CD8-PE (BD Biosciences), CD11b-PE (Biolegend), F4/80-FITC (eBioscience), NK1.1 (Biolegend) and CD19-PC7 (BD Pharmingen). Cells were measured with an FC 500 Coulter Beckman. Gating strategy is shown in Supplementary Fig. 6 . RNA isolation and gene expression Total RNA was isolated from adipose tissue using TRIzol (Invitrogen, Carlsbad, CA), according to the manufacturer’s instructions. RNA was reverse-transcribed (iScript cDNA Synthesis Kit, Bio-Rad Laboratories). Reverse transcription–PCR was performed using specific primers (see Supplementary Table 1 ), power SYBR green master mix (Applied Biosystems, Foster City, CA) using the Step-one Real-Time PCR system (Applied Biosystems). For mice samples, we used 36B4 as a housekeeping gene to correct the values. F4/80 , MCP-1 , and CD68 and human IL-37 were analysed. For human samples, we used B2M as a housekeeping gene. Primers sequences are shown in Table 2 . Table 2 Primers used for quantitative real-time PCR analysis. Full size table Western blot analysis For mouse and human samples, lysates were prepared using a lysis buffer (50 mM Tris (pH7.4), 150 mM NaCl, 2 mM EDTA,1% Nonidet P-40, 50 mM NaF and 0.25% sodium deoxycholate with PhosStop Phosphatase-Inhibitor Cocktail tablet (Roche) and complete, EDTA-free protease-inhibitor cocktail tablet (Roche). The homogenate was centrifuged at 4 °C for 10 min at 18,000 r.c.f. and the supernatant was used for western blot analysis. Equal amounts of protein, as determined by a BCA protein assay (Thermo FisherScientific, Rockford, IL) were separated using a polyacrylamide SDS–PAGE gel. After SDS–PAGE, proteins were transferred to a nitrocellulose membrane using a Trans-Blot Turbo Transfer System (Biorad) following the manufacturer’s instructions. The membrane was blocked with 5% (wt/vol) milk powder in Tris-buffered saline (TBS)/Tween 20 for 1 h at room temperature followed by incubation overnight at 4 °C with an IL-37 antibody (R&D systems), AMPK or phospho-AMPK antibodies (Cell Signaling) in 5% (wt/vol) milk powder/TBS/Tween 20 or with an actin antibody (Sigma-Aldrich, St Louis, MO) in 5% milk powder in TBS/Tween 20. After overnight incubation, the blots were incubated with horseradish peroxidase (HRP)-conjugated secondary antibodies at a dilution of 1:5,000 in 5% (wt/vol) milk powder in TBS/Tween 20 for 1 h at room temperature and subsequently developed with ECL plus (Thermo Scientific) according to the manufacturer’s instructions. Bands were visualized using a ChemiDoc System (Biorad) and quantified using Image lab software (Biorad). From human HepG2 hepatoma cells, proteins were separated under reducing conditions on 8% bis-acrylamide gels. Proteins were then blotted on polyvinylidene difluoride membranes. Blocking, incubation steps with first/second antibodies, and washing was performed using a SNAP i.d. protein detection system according to the manufacturer’s instructions (Millipore). The following antibodies have been used: anti-phospho-IRS1 (Tyr941), anti-IRS1, anti phospho-Akt (Ser473), anti pan-Akt, anti-GAPDH (all Cell Signaling), anti-rabbit immunoglobulins/HRP and anti-mouse immunoglobulins/HRP (both Dako). Bands were visualized using a chemoluminescent substrate and chemoluminescent films (GE Healthcare). Uncropped images of immunoblottings are shown in Supplementary Fig. 12 . Cell culture Human HepG2 hepatoma cells were seeded in 10-cm culture tissue plates. Cells were transfected with either IL-37-specific or scrambled siRNAs using siPORT NeoFX transfection reagent (Ambion). Cells were starved overnight in DMEM/0.25% fat-free BSA. The next morning, cultures were stimulated with 25 ng ml −1 TNF-α for 10 min or 5 μg ml −1 tunicamycin for 4 h, respectively. Thereafter, HepG2s were stimulated with 10 nM insulin for 5 min. The media were decanted, plates were immediately placed on ice and washed with ice-cold PBS containing phosphatase inhibitors. Protein extraction was performed with M-PER protein extraction reagents containing protease and phosphatase inhibitors according to the manufacturer’s instructions (Pierce). Human SGBS cells were differentiated with or without recIL-37 (10 ng ml −1 ). Differentiation was done as previously described [62] . In short, the differentiation was initiated by incubating the cells in medium (DMEM/F12, Gibco Life Technologies, Bleiswijk, The Netherlands) without serum in the presence of 2 μmol l −1 rosiglitazone, 25 nmol l −1 dexamethasone, 0.5 mmol l −1 methylisobutylxanthine, 0.1 μmol l −1 cortisol, 0.01 mg ml −1 transferrin, 0.2 nmol l −1 triiodothyronine (all from Sigma-Aaldrich, Zwijndrecht, The Netherlands) and 20 nmol l −1 insulin. Four days later, the medium was only enriched by 0.1 μmol l −1 cortisol, 0.01 mg ml −1 transferrin, 0.2 nmol l −1 triiodothyronine and 20 nmol l −1 insulin. After 2 weeks, light microscopy pictures were taken at magnification of × 20 and mRNA was isolated as described. Microarray analysis RNA isolated from adipose tissue from HFD-fed animals was used for microarray analysis ( n =4 animals per group). RNA quality was determined by analysis on the Agilent 2100 Bio-analyser, and all samples had an RNA Integrity Number (RIN) score >8. The Ambion WT Expression kit (Life Technologies) in conjunction with the Affymetrix GeneChip WT Terminal Labelling kit (Affymetrix, Santa Clara, CA) was used to prepare labelled complementary DNA from 100 ng of total RNA. Samples were hybridized on Affymetrix GeneChip Mouse Gene 1.0 ST arrays. Differences in gene expression between WT and IL-37tg -derived epididymal tissue were determined using gene set enrichment analysis. The Enrichment Map plug-in for Cytoscape was used for visualization and interpretation of the gene set enrichment analysis results. The cut-off values were P <0.01. Statistical analysis Data are shown as the mean±s.e.m. Differences between groups were statistically analysed using Student’s t test, and differences among the four groups were analysed with analysis of variance followed by post-hoc Bonferroni tests in Graphpad Prism 5.0. When necessary, results were log-transformed to normalize the data. A P -value<0.05 was considered significant. Accession codes: Microarray data have been deposited in GEO repository under accession code GSE58952 . How to cite this article: Ballak, D. B. et al. IL-37 protects against obesity-induced inflammation and insulin resistance. Nat. Commun. 5:4711 doi: 10.1038/ncomms5711 (2014).